Tailoring gadolinium-doped ceria-based solid oxide fuel cells to achieve 2 W cm−2at 550 °C Low-temperature operation is necessary for next-generation solid oxide fuel cells due to the wide variety of their applications. However, significant increases in the fuel cell losses appear in the low-temperature solid oxide fuel cells, which reduce the cell performance. To overcome this problem, here we report Gd 0.1 Ce 0.9 O 1.95 -based low-temperature solid oxide fuel cells with nanocomposite anode functional layers, thin electrolytes and core/shell fibre-structured Ba 0.5 Sr 0.5 Co 0.8 Fe 0.2 O 3− δ -Gd 0.1 Ce 0.9 O 1.95 cathodes. In particular, the report describes the use of the advanced electrospinning and Pechini process in the preparation of the core/shell-fibre-structured cathodes. The fuel cells show a very high performance of 2 W cm −2 at 550 °C in hydrogen, and are stable for 300 h even under the high current density of 1 A cm −2 . Hence, the results suggest that stable and high-performance solid oxide fuel cells at low temperatures can be achieved by modifying the microstructures of solid oxide fuel cell components. Low-temperature solid oxide fuel cells (LT-SOFCs) have attracted significant attention because of their potential long-term stability, shorter start-up times and economic competitiveness for a large number of applications, such as small-scale portable devices, auxiliary power units for automobiles and large distributed power generation systems [1] , [2] , [3] , [4] , [5] . However, significant increases in the fuel cell losses, especially ohmic and activation losses, appear in the LT-SOFCs, which reduce the cell performance. The ohmic and activation losses are mainly due to oxygen ion transport through the electrolyte and the slow reaction kinetics on surfaces of the electrodes, respectively. The approaches to reducing such losses at low temperatures can be easily found in the equations for forward current density and ohmic resistance [6] : using electrolyte materials with fast ionic conductivity at low temperatures, reducing electrolyte thickness, increasing the reactant concentration and the number of possible reaction sites and decreasing the activation barrier. A number of electrolyte materials have been developed to reduce ohmic resistance at low temperatures. Among these materials, ceria-based materials, especially gadolinium-doped ceria (GDC), have been considered strong candidates for LT-SOFC electrolytes due to their high ionic conductivity at intermediate and low operating temperatures. However, the ceria-based electrolyte can introduce electronic conduction by partially reducing CeO 2 to CeO 2− δ at low oxygen partial pressures, which restricts the reduction of the electrolyte thickness [7] , [8] , [9] . For that reason, studies on the fabrication of thin electrolytes have focused on yttria-stabilized zirconia, which has been widely used as an electrolyte material at high temperatures, rather than the ceria-based electrolytes [10] , [11] , [12] , [13] . When using the thin ceria-based electrolytes, buffer layers should be applied to protect the materials from reduction by preventing contact with the reducing gas [14] , [15] . The former often uses expensive deposition devices, such as pulsed laser deposition [12] that many researchers have chosen to prepare the thin film, and the latter requires complex cell fabrication processes and has the possibility of thermal expansion mismatch between the GDC and the buffer layers. The dip-coating method is one of the most cost-effective wet-coating processes [16] , [17] , [18] , but accurate thickness control and thin layer fabrication are limited. Accordingly, we attempted to deposit the GDC thin electrolyte by controlling the compositions of the electrolyte slurries in the dip-coating method in order to reduce the ohmic loss. To reduce the activation loss, the number of possible reaction sites has been increased by modifying the electrode microstructures or by introducing anode functional layers (AFLs). An AFL has been applied to the anode side for the purpose of increasing triple phase boundary (TPB) sites where reactants, electrolyte and catalyst are in contact [19] , [20] . In the cathode part, the perovskite-type materials, such as Sm 0.5 Sr 0.5 CoO 3− δ (SSC) [21] and La 0.6 Sr 0.4 Co 1− x Fe x O 3− δ (LSCF) [22] have been mainly used for low-temperature operation. Shao and Haile recently reported Ba 0.5 Sr 0.5 Co 0.8 Fe 0.2 O 3− δ (BSCF) as a new cathode material for LT-SOFCs [23] , and as a consequence, a number of studies have focused on the physical and electrochemical properties of the BSCF cathode depending on its microstructure and composition, as the reaction kinetics on the surface of inorganic materials are specific to their compositions and configurations [24] , [25] , [26] , [27] , [28] , [29] , [30] , [31] , [32] , [33] . In recent years, we confirmed that the nanocomposite Ni-GDC AFL [34] and the core/shell fibre structured BSCF-GDC cathode have positive influences on the cell performance at low temperatures. In particular, the advanced electrospinning & Pechini (AE&P) process to fabricate the inorganic core/shell fibres is described here by preparing the core/shell-fibre-structured BSCF-GDC cathode, which has many advantages, such as direct use of inorganic particles including ceramic oxides as precursors, decreased shrinkage rate of the mats, simplification of the entire electrospinning process and time saving in the preparation of inorganic fibres. Despite the numerous studies on each part (anode, cathode and electrolyte), high-performance LT-SOFCs, especially ceria-based LT-SOFCs [35] , [36] , [37] , [38] , have been rarely reported with few exceptions: Wachsman et al. [4] reported 2 W cm −2 at 650 °C in a cell with an Er 0.4 Bi 1.6 O 3 -Gd 0.1 Ce 0.9 O 1.95 bilayer and a bismuth ruthenate bismuth oxide (BRO7-ESB) composite cathode, Yan et al. reported ~1 W cm −2 maximum power density at 550 °C using a La 0.9 Sr 0.1 Ga 0.8 Mg 0.2 O 3− δ (LSGM) electrolyte with a Ce 0.8 Sm 0.2 O 2− δ (SDC) buffer layer [39] and Choi et al. [40] and Park et al. [41] recently reported over 1.2 W cm −2 at 550 °C in a cell with a PrBa 0.5 Sr 0.5 Co 1.5 Fe 0.5 O 5+ δ (PBSCF05) cathode. Here, we report an original cell design, the core/shell-fibre-structured BSCF-GDC cathode | thin GDC electrolyte | nanocomposite Ni-GDC AFL | Ni-GDC anode fuel cell to achieve high and stable performance GDC-based LT-SOFCs. 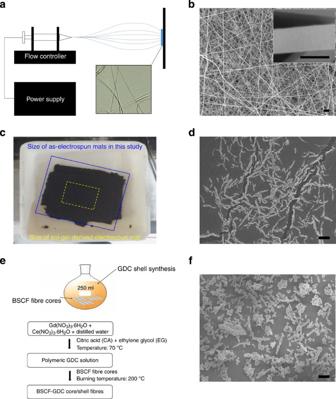Figure 1: Fabrication and scanning electron microscopy (SEM) images of the BSCF-GDC core/shell fibre (a), advanced electrospinning step based on dispersed particles and an optical image of the as-electrospun Ba0.5Sr0.5Co0.8Fe0.2O3−δ(BSCF) core fibre, (b), SEM image of the as-electrospun BSCF core fibre (the inset represents the SEM image at high magnification), scale bars, 1 μm and 100 nm (inset), (c), colour photograph of the BSCF core-fibre mats calcined at 500 °C, (d), SEM image of the BSCF core fibres calcined at 500 °C, scale bar: 10 μm, (e), flow chart of Pechini step, (f), SEM image of the Ba0.5Sr0.5Co0.8Fe0.2O3−δ-Gd0.1Ce0.9O1.95(BSCF-GDC) core/shell fibres calcined at 600 °C after Pechini step, scale bar, 10 μm. The GDC-based LT-SOFCs exhibit an outstanding performance of approximately 2 W cm −2 at 550 °C, which is stable for 300 h even under the high current density of 1 A cm −2 ( Supplementary Figure 1 represents the apparatus for anode-supported cell tests in this study). As a result, it demonstrates that modifying the microstructures of solid oxide fuel cell components is necessary for low-temperature operation, and the GDC-based LT-SOFCs with the nanocomposite AFL, thin electrolytes and core/shell fibre structured BSCF-GDC cathodes can be promising to achieve the high and stable performance at low temperatures. BSCF-GDC core/shell fibres We have developed the fibrous cathode via the advanced electrospinning (AE). In our previous study, the electrospun La 0.6 Sr 0.4 Co 0.2 Fe 0.8 -Gd 0.1 Ce 0.9 O 1.95 (LSCF-GDC) cathode with the well-connected fibrous networks and the high porosity reduced the activation loss, decreasing the resistances with respect to charge transfer, oxygen surface exchange and gas diffusion [42] , [43] , [44] . To upgrade the fibrous cathode, we recently developed the core/shell fibre structured BSCF-GDC cathode via the AE&P process. Figure 1 shows the whole processes for the fabrication of the BSCF-GDC core/shell fibres via the AE&P process, including their optical and scanning electron microscopy (SEM) images. In the first step, the electrospun PVP-BSCF mixtures formed hair-like nanowires ( Fig. 1a ). The diameter of the nanowire was about 100 nm, which was tangled over one another to produce a fine web ( Fig. 1b ). The sol-gel-derived electrospun mats typically show significant shrinkage as indicated by the yellow dot box in Fig. 1c , which limits the application of ceramic nanowires by generating strong stress during the calcination process [45] . However, the BSCF core fibre mats rarely shrank during the calcination at 500 °C, and the fibrous shape also remained in the calcined BSCF core fibres ( Fig. 1d ). Besides, Pechini synthesis ( Fig. 1e ) for covering the BSCF core fibres with the GDC nanoparticles is accompanied with vigorous stirring and weak explosion, but Fig. 1f clearly shows that the BSCF-GDC core/shell fibres calcined at 600 °C still retain the fibrous shapes. The formation of the BSCF-GDC core/shell fibres via the AE&P process can be conjectured based on the following: (1) as-synthesized core/shell fibres had only the perovskite structures corresponding to the BSCF, while the perovskite structures of the BSCF as well as cubic fluorite structures of the GDC appeared after calcination at 600 °C ( Fig. 2a ) and (2) the difference in the weight losses between the BSCF core fibres (10%) and the BSCF-GDC core/shell fibres (20%) could be mainly caused by the polymers included in the GDC shell particles ( Fig. 2b ). More specific confirmation of the core/shell fibre structures is discussed in the next section. Figure 1: Fabrication and scanning electron microscopy (SEM) images of the BSCF-GDC core/shell fibre ( a ), advanced electrospinning step based on dispersed particles and an optical image of the as-electrospun Ba 0.5 Sr 0.5 Co 0.8 Fe 0.2 O 3−δ (BSCF) core fibre, ( b ), SEM image of the as-electrospun BSCF core fibre (the inset represents the SEM image at high magnification), scale bars, 1 μm and 100 nm (inset), ( c ), colour photograph of the BSCF core-fibre mats calcined at 500 °C, ( d ), SEM image of the BSCF core fibres calcined at 500 °C, scale bar: 10 μm, ( e ), flow chart of Pechini step, ( f ), SEM image of the Ba 0.5 Sr 0.5 Co 0.8 Fe 0.2 O 3− δ -Gd 0.1 Ce 0.9 O 1.95 (BSCF-GDC) core/shell fibres calcined at 600 °C after Pechini step, scale bar, 10 μm. 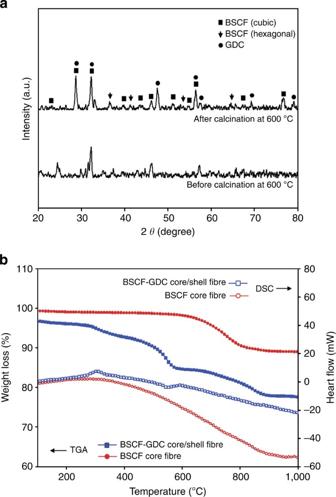Figure 2: X-ray diffractometre (XRD) patterns and thermogravimetric analysis (TGA)/differential scanning calorimeter (DSC) curves of the BSCF-GDC core/shell fibre. (a), XRD patterns of the Ba0.5Sr0.5Co0.8Fe0.2O3−δ-Gd0.1Ce0.9O1.95(BSCF-GDC) core/shell fibres before and after calcination at 600 °C, and (b), TGA/DSC curves of the BSCF core fibres and BSCF-GDC core/shell fibres obtained before the calcination process. The TGA/DSC was measured in a temperature range from 100 to 1,000 °C in air atmosphere. Full size image Figure 2: X-ray diffractometre (XRD) patterns and thermogravimetric analysis (TGA)/differential scanning calorimeter (DSC) curves of the BSCF-GDC core/shell fibre. ( a ), XRD patterns of the Ba 0.5 Sr 0.5 Co 0.8 Fe 0.2 O 3− δ -Gd 0.1 Ce 0.9 O 1.95 (BSCF-GDC) core/shell fibres before and after calcination at 600 °C, and ( b ), TGA/DSC curves of the BSCF core fibres and BSCF-GDC core/shell fibres obtained before the calcination process. The TGA/DSC was measured in a temperature range from 100 to 1,000 °C in air atmosphere. Full size image Confirmation of the core/shell fibre structures The BSCF-GDC core/shell fibre structures were confirmed by using SEM and high-resolution transmission electron microscopy (HRTEM) as shown in Fig. 3 . The BSCF core fibre was approximately 1 μm in diameter, and BSCF particles with 100–200-nm size were closely connected to each other to form the fibres ( Fig. 3a ). After the covering process, the diameters of the fibres slightly increased to 1.2–1.5 μm, which could be caused by the polymeric Gd and Ce nanoparticles surrounding the BSCF core fibre ( Fig. 3b ). Compared with the BSCF core fibre in Fig. 3a , the fibres in Fig. 3b had smoother surfaces. The pores existing between the linked BSCF particles in the core fibres would be filled by the synthesized polymeric nanoparticles, which can demonstrate that the polymeric nanoparticles were wrapped up around the core fibres. 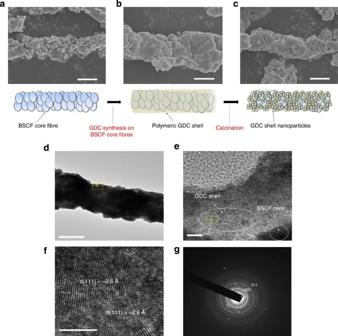Figure 3: Scanning electron microscopy (SEM) images including schematic diagrams and high-resolution transmission electron microscopy (HRTEM) images. (a), SEM image of the Ba0.5Sr0.5Co0.8Fe0.2O3−δ(BSCF) core fibre after calcination at 500 °C, (b), SEM image of the Ba0.5Sr0.5Co0.8Fe0.2O3−δ-Gd0.1Ce0.9O1.95(BSCF-GDC) core/shell fibre right after polymeric synthesis, and (c), SEM image of the BSCF-GDC core/shell fibre after calcination at 600 °C, scale bar, 1 μm (a,bandc). (d), transmission electron microscopy (TEM) image of the BSCF-GDC rod with different brightness, displaying the shape characteristics of the fibres, scale bar, 1 μm, (e), HRTEM image from box 1 ind, showing the bright Gd0.1Ce0.9O1.95(GDC) shell particles attached to dark BSCF core fibres, scale bar, 10 nm, (f), HRTEM image from box 2 ine, showing the random arrangement of the GDC lattices, scale bar: 5 nm, and (g), the electron diffraction pattern fromf. Figure 3c shows the polymeric Gd and Ce nanoparticles around the BSCF fibre cores were decomposed and changed into the metal oxide, GDC, after calcination at 600 °C. Small pores appeared again on the surfaces of the BSCF core fibre, and the fibre thickness also decreased after the decomposition of the polymers. To precisely observe the pores and the morphologies of the BSCF-GDC core/shell fibres in Fig. 3c , magnified SEM images were collected using energy-dispersive X-ray spectroscopy (EDX) point measurements ( Supplementary Fig. 2 and Supplementary Table 1 ), which clearly show that the GDC nanoparticles tightly covered the BSCF fibre core. The EDX point measurement indicated not only the elements in the BSCF fibre core but also the Gd and Ce elements, which supports the above discussion. Considering the fibre cores were prepared using BSCF particles, the existence of Gd and Ce elements on the fibre means the GDC nanoparticles cover the BSCF core fibre. Furthermore, the amount of each element corresponded to the stoichiometric ratio of Ba 0.5 Sr 0.5 Co 0.8 Fe 0.2 O 3− δ and Gd 0.1 Ce 0.9 O 1.95 at the time the materials were fabricated and synthesized. Figure 3d–g show transmission electron microscopy (TEM) and HRTEM images of the BSCF-GDC core/shell fibre after calcination at 600 °C. The BSCF-GDC core/shell fibre had a diameter of 1 μm, which was similar to the size observed in the SEM images ( Fig. 3d ). Figure 3e shows the HRTEM image obtained from box 1 in Fig. 3d , which clearly shows that the bright nanoparticles were attached around the dark fibre core. Figure 3f,g show the magnified image from box 2 in Fig. 3e and the electron diffraction image obtained from Fig. 3f . The bright nanoparticles had a d-spacing value of approximately 2.6 Å. The electron diffraction patterns and Debye–Scherrer rings of the bright nanoparticles can be consistently indexed as those of GDC with a cubic fluorite structure [46] , [47] , which demonstrates that the bright GDC nanoparticles attached around the BSCF fibre core and the core/shell fibres can be prepared simply via the AE&P process without their structures collapsing during the process. Figure 3: Scanning electron microscopy (SEM) images including schematic diagrams and high-resolution transmission electron microscopy (HRTEM) images. ( a ), SEM image of the Ba 0.5 Sr 0.5 Co 0.8 Fe 0.2 O 3− δ (BSCF) core fibre after calcination at 500 °C, ( b ), SEM image of the Ba 0.5 Sr 0.5 Co 0.8 Fe 0.2 O 3− δ -Gd 0.1 Ce 0.9 O 1.95 (BSCF-GDC) core/shell fibre right after polymeric synthesis, and ( c ), SEM image of the BSCF-GDC core/shell fibre after calcination at 600 °C, scale bar, 1 μm ( a , b and c ). ( d ), transmission electron microscopy (TEM) image of the BSCF-GDC rod with different brightness, displaying the shape characteristics of the fibres, scale bar, 1 μm, ( e ), HRTEM image from box 1 in d , showing the bright Gd 0.1 Ce 0.9 O 1.95 (GDC) shell particles attached to dark BSCF core fibres, scale bar, 10 nm, ( f ), HRTEM image from box 2 in e , showing the random arrangement of the GDC lattices, scale bar: 5 nm, and ( g ), the electron diffraction pattern from f . Full size image Symmetrical cell tests on the core/shell fibre electrodes The conventional and core/shell fibre structured BSCF-GDC electrodes were applied to the symmetrical cells. The electrode thicknesses were approximately 10 μm in both cells ( Supplementary Fig. 3 ). First, Fig. 4a shows that good linearity of the area-specific resistance (ASR) of the cathodes versus the reciprocal temperature was observed over the operating temperature range from 450 to 600 °C, and the derived activation energies were ~105 and ~114 kJ mol −1 in the core/shell fibre-structured BSCF-GDC cathode and the conventional BSCF-GDC cathode, respectively, which are almost similar to the oxygen surface exchange step (113±11 kJ mol −1 ) [23] . This result suggests that oxygen surface exchange is still the rate-limiting step at low temperatures in both electrodes. The cathode ASR was determined from raw impedance plots, where the high-frequency offset is due to the electrolyte resistance and the radius of the impedance arc is due to the cathode resistance. The ASR of the core/shell fibre structured BSCF-GDC cathode is noticeably lower than that of the conventional BSCF-GDC cathode: 0.552 Ω cm 2 at 550 °C in the core/shell fibre-structured cathode and 1.115 Ω cm 2 at the same temperature in the conventional cathode ( Fig. 4b ). The results are much higher than the ASR (~0.19 Ω cm 2 at 550 °C on about 20 μm-thick electrodes) reported by Shao and Heile [23] , but it may result from the thinner electrode thickness (~10 μm) in both cells [23] , [48] . Table 1 shows the comparison of the ASRs and summit frequencies between the two electrodes at different temperatures, obtained from the raw impedance spectra in Supplementary Fig. 4 . The cathode ASRs for both types of the electrodes were greatly increased from 500 °C. We believe that it is largely associated with the nature of the BSCF material. However, the limit of this material property was improved by the structural modification in this study. The ASRs of the conventional BSCF-GDC electrode were changed from 1.115 to 3.361 Ω cm 2 and from 3.361 to >12,000 Ω cm 2 with a decrease in the temperature from 550 to 500 °C and from 500 to 450 °C, while the ASRs of the BSCF-GDC core/shell fibre electrode decreased from 0.552 to 1.284 Ω cm 2 and from 1.284 to 4.717 Ω cm 2 with decreases in the temperatures from 550 to 500 °C and from 500 to 450 °C, respectively. Shao and Haile [23] reported that increase in the area over which the surface exchange could occur, for example, an increase in the cathode thickness results in decreases in the ASR without a change in the activation energy. Despite the same thickness of both electrodes ( Supplementary Fig. 3 ), a significant decrease in the ASR of the core/shell fibre-structured BSCF-GDC cathode demonstrates that the area over which the surface exchange occurs can be significantly increased by the core/shell fibre structures modified in this study. Furthermore, low-frequency contributions with respect to the oxygen surface exchange occur in both electrodes, which support the claim that the core/shell fibre electrodes with lower ASR have better oxygen surface exchange kinetics. Here, two contributions to this improvement can be largely expected: large specific surface area and morphological characteristics of the core/shell fibre-structured BSCF-GDC cathode. 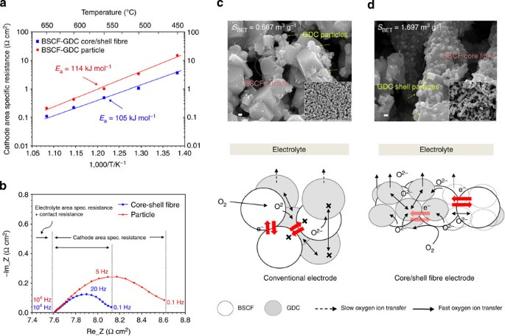Figure 4: ASR of the symmetrical cells under air. (a), ASR of the conventional and core/shell fibre Ba0.5Sr0.5Co0.8Fe0.2O3−δ-Gd0.1Ce0.9O1.95(BSCF-GDC) electrodes as a function of temperature, and (b), a typical impedance spectrum, as obtained from the two electrodes with a thickness of about 10 μm, symmetrical cell at 550 °C (raw impedance data have been multiplied by the cathode area, 0.785 cm2, so that the cathode ASR corresponds directly to the diameter of the arc associated with the cathode response). Surface scanning electron microscopy (SEM) images of the electrodes applied to the symmetrical cells: (c), conventional BSCF-GDC particle electrode (the inset represents the SEM image at low magnification), scale bars, 100 nm and 1 μm (inset), and (d), the core/shell fibre structured BSCF-GDC electrode (the inset represents the SEM image at low magnification), scale bar: 100 nm and 1 μm (inset). The corresponding schematic diagrams of the electrochemical reactions on the BSCF-GDC particle electrode and the BSCF-GDC core/shell fibre electrode: fast oxygen ion transfer from the electrode into the electrolyte occurs in the BSCF-GDC core/shell fibre electrode due to well-distributed Gd0.1Ce0.9O1.95(GDC) particles and well-connected BSCF-GDC core fibres, while the BSCF-GDC particle electrode may suffer from the slow oxygen ion transfer due to random distribution of the GDC and BSCF particles. Figure 4c,d certainly prove the former, indicating the larger specific surface area ( S BET ) of 1.697 m 2 g −1 in the BSCF-GDC core/shell fibres than the S BET of 0.667 m 2 g −1 in the conventional BSCF-GDC particles ( Supplementary Fig. 5 ). The latter can be explained using the SEM images that correspond to the schematic diagrams of both the particle and core/shell fibre electrodes in Fig. 4c,d . The differences in the microstructures between the conventional and core/shell fibre BSCF-GDC electrodes are clearly shown in the insets from Fig. 4c,d . For the conventional BSCF-GDC electrode, the GDC particles with 100–200 nm sizes were irregularly and sparsely attached to the large BSCF particles with 500–800 nm sizes ( Fig. 4c ). In addition, the GDC particles that support oxygen ion transfer should be attached to the BSCF particles, but they were coupled not only to the BSCF particles but also to the GDC particles. This combination of GDC particles may degrade the cathodic properties of the BSCF-GDC electrode. Interestingly, the core/shell fibre-structured BSCF-GDC electrode via the AE&P process maintained their core/shell fibre structures even after application in the electrode ( Fig. 4d ). The GDC shell particles with regular 100-nm sizes were uniformly attached around the BSCF fibre cores with diameters of approximately 1 μm. The BSCF fibre cores act as the primary structure for transferring electrons and oxygen ions by being closely connected. The GDC shell nanoparticles play a role in facilitating oxygen ion transfer because they are attached to the BSCF fibre cores. In addition, the homogeneous distribution of the GDC shell particles on the BSCF core fibres may promote oxygen ion transfer from the BSCF core fibres and the neighbour GDC nanoparticles to the electrolyte. This schematic diagram corresponds well to the SEM images of the core/shell fibre-structured BSCF-GDC electrode in Fig. 4d . Further analysis of the ASRs in the BSCF-GDC core/shell fibre electrode and La 0.6 Sr 0.4 Co 0.2 Fe 0.8 O 3− δ -Gd 0.1 Ce 0.9 O 1.95 (LSCF-GDC) single-fibre electrode is represented in Supplementary Discussion with Supplementary Fig. 6 and Supplementary Table 2 . Figure 4: ASR of the symmetrical cells under air. ( a ), ASR of the conventional and core/shell fibre Ba 0.5 Sr 0.5 Co 0.8 Fe 0.2 O 3− δ -Gd 0.1 Ce 0.9 O 1.95 (BSCF-GDC) electrodes as a function of temperature, and ( b ), a typical impedance spectrum, as obtained from the two electrodes with a thickness of about 10 μm, symmetrical cell at 550 °C (raw impedance data have been multiplied by the cathode area, 0.785 cm 2 , so that the cathode ASR corresponds directly to the diameter of the arc associated with the cathode response). Surface scanning electron microscopy (SEM) images of the electrodes applied to the symmetrical cells: ( c ), conventional BSCF-GDC particle electrode (the inset represents the SEM image at low magnification), scale bars, 100 nm and 1 μm (inset), and ( d ), the core/shell fibre structured BSCF-GDC electrode (the inset represents the SEM image at low magnification), scale bar: 100 nm and 1 μm (inset). The corresponding schematic diagrams of the electrochemical reactions on the BSCF-GDC particle electrode and the BSCF-GDC core/shell fibre electrode: fast oxygen ion transfer from the electrode into the electrolyte occurs in the BSCF-GDC core/shell fibre electrode due to well-distributed Gd 0.1 Ce 0.9 O 1.95 (GDC) particles and well-connected BSCF-GDC core fibres, while the BSCF-GDC particle electrode may suffer from the slow oxygen ion transfer due to random distribution of the GDC and BSCF particles. Full size image Table 1 Symmetrical cell tests. Full size table First- and second-generation GDC-based LT-SOFCs On the basis of the improved electrochemical properties of the core/shell fibre-structured BSCF-GDC cathode, we prepared two types GDC-based LT-SOFCs: first generation—the core/shell fibre structured BSCF-GDC (~24 μm) | GDC (~9 μm) | Ni-GDC (800 μm) fuel cell ( Fig. 5a ) and second generation—the core/shell-fibre-structured BSCF-GDC (~30 μm) | GDC (~5 μm) | nanocomposite Ni-GDC AFL (~10 μm) | Ni-GDC (~800 μm) fuel cell ( Fig. 5b ). As shown in Fig. 5a,b , the core/shell fibre-structured BSCF-GDC cathode via the AE&P process was reproducible in terms of their structures. The first and second generation cells were 0.908 and 0.923 V in the open circuit voltage (OCV), which is acceptable for GDC-based cells ( Fig. 5c ). Compared with approximately 0.65–0.7 W cm −2 at 550 °C based on Ni-SDC | SDC (20 μm) | BSCF cells reported by Shao and Haile [23] and 0.86 W cm −2 at 550 °C based on Ni-GDC | GDC (10 μm) | sol-gel-derived BSCF cells reported by Liu et al. [31] , the maximum power densities were dramatically increased in both first and second generation cells, showing 1.14 and 1.97 W cm −2 at 550 °C, respectively. The first generation cell had an approximately 9-μm-thick electrolyte, which is similar to the thickness in the study of Liu et al. [31] . The fact that, despite the similar electrolyte thickness, higher peak power densities appeared in the first generation cell substantiates the improved performance of the core/shell fibre cathode in terms of oxygen surface exchange. In particular, the second generation cell is worthy to note that the cell performance of approximately 2 W cm −2 at 550 °C has not been reported yet for LT-SOFCs fabricated using cost-effective and straightforward processes. Furthermore, the cell performance of 0.84 W cm −2 at 450 °C in Table 2 and Supplementary Fig. 7 can match the three-dimensional nanostructured bilayer solid oxide fuel cell with 1.3 W cm −2 at 450 °C via atomic layer deposition recently reported by An et al. [14] . The marked difference in the peak power density between first and second generation cells can be explained from Fig. 5d . First, ASR ohmic of the second generation cell was significantly decreased from 0.11 to 0.05 Ω cm 2 by the reduction of the electrolyte thickness from 9 to 5 μm. Although Steele reported that the minimum thickness for dense impermeable films is approximately 10–15 μm in terms of reliable mass production using relatively cheap ceramic fabrication routes [7] , in this study, it was possible to obtain only 5-μm-thick electrolyte using the cost-effective dip-coating process for reliably mass production. The helium permeability of the GDC thin film was 2.06 × 10 −9 mol m −2 s −1 Pa −1 at 0.25 Mpa ( Supplementary Fig. 8 ), which indicates that the film is sufficiently gas tight as the SOFC electrolyte [49] . Second, as shown in the SEM images ( Fig. 5b ), the nanocomposite AFL of the second generation cell would reduce the ASR electrode (the sum of the anode and cathode contributions) from 0.059 to 0.043 Ω cm 2 at 550 °C, based on the contribution of the core/shell fibre BSCF-GDC cathode as referred to earlier. The positive effects of the nanocomposite AFL on the electrochemical properties in the anode side were already described in our previous study [34] . Moreover, we could avoid the constriction effect that makes the actual ohmic resistance higher than the calculated one based on the electrolyte thickness by controlling the AFL thickness. Considering the constrictions within the flow of current through the electrolyte occur at the triple phase boundary at the electrode–electrolyte interface and create the competition between mass and electronic transport losses [50] , [51] , [52] , [53] , in our previous study, the constriction resistance could result from the 23-μm-thick and dense nanocomposite AFL (ASR ohmic : 0.11 Ω cm 2 on the 7-μm-thick electrolyte) that can limit the mass transport in the anode side. Thus, we attempted to reduce the AFL thickness, and consequently, the reduction in the AFL thickness into 10 μm (ASR ohmic : 0.05 Ω cm 2 on the 5-μm-thick electrolyte) was effective for preventing the constriction effects. The difference in the cathode thickness may also have influences on the ASR electrode , but it cannot be exactly confirmed in this study due to the different cell configurations between the first and second generation cells. However, we assume that the AFL contributions to decrease in the electrode resistance may be offset by increase in the resistance of the thick cathode because a slight drop in the ASR electrode , despite the nanocomposite AFL and thicker cathode from 24 to 30 μm ( Fig. 5a,b ), occurred in the second generation cell. Sasaki et al. [48] reported that the cathode thickness more than about 25 μm increased both the ohmic and electrode resistance, which can support our assumptions. Therefore, the optimization of the BSCF-GDC cathode thickness should be required to achieve higher performance than our present results. 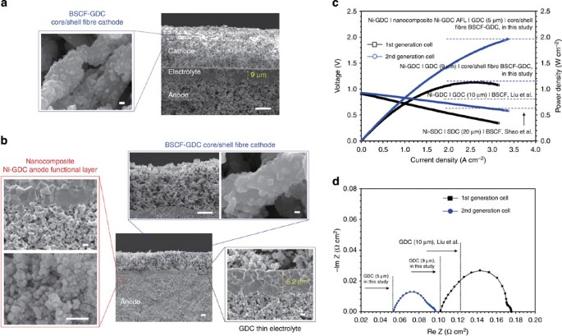Figure 5: Scanning electron microscopy (SEM) images and performances on the first and second generation cells. (a), SEM image of the first generation cell in configuration of the core/shell fibre structured Ba0.5Sr0.5Co0.8Fe0.2O3−δ-Gd0.1Ce0.9O1.95(~24 μm) | Gd0.1Ce0.9O1.95(~9 μm) | Ni-Gd0.1Ce0.9O1.95(800 μm), Scale bar, first generation cell image—10 μm and core/shell fibre image—100 nm, (b), SEM image of the second generation cell in configuration of the core/shell-fibre-structured Ba0.5Sr0.5Co0.8Fe0.2O3−δ-Gd0.1Ce0.9O1.95(~30 μm) | Gd0.1Ce0.9O1.95(~5 μm) | nanocomposite Ni-Gd0.1Ce0.9O1.95anode functional layer (AFL) (~10 μm) | Ni-Gd0.1Ce0.9O1.95(~800 μm), Scale bar, second generation cell image—10 μm, AFL images—1 μm (top) and 100 nm (bottom), core/shell fibre images—10 μm (left) and 100 nm (right), and electrolyte image—1 μm, (c), cell voltage and power density as functions of current density and (d), a typical impedance spectrum measured under open circuit conditions. The tests were carried out at 550 °C. Air was supplied to the cathode (300 ml min−1) and H2was supplied to the anode (80 ml min−1). Figure 5: Scanning electron microscopy (SEM) images and performances on the first and second generation cells. ( a ), SEM image of the first generation cell in configuration of the core/shell fibre structured Ba 0.5 Sr 0.5 Co 0.8 Fe 0.2 O 3− δ -Gd 0.1 Ce 0.9 O 1.95 (~24 μm) | Gd 0.1 Ce 0.9 O 1.95 (~9 μm) | Ni-Gd 0.1 Ce 0.9 O 1.95 (800 μm), Scale bar, first generation cell image—10 μm and core/shell fibre image—100 nm, ( b ), SEM image of the second generation cell in configuration of the core/shell-fibre-structured Ba 0.5 Sr 0.5 Co 0.8 Fe 0.2 O 3− δ -Gd 0.1 Ce 0.9 O 1.95 (~30 μm) | Gd 0.1 Ce 0.9 O 1.95 (~5 μm) | nanocomposite Ni-Gd 0.1 Ce 0.9 O 1.95 anode functional layer (AFL) (~10 μm) | Ni-Gd 0.1 Ce 0.9 O 1.95 (~800 μm), Scale bar, second generation cell image—10 μm, AFL images—1 μm (top) and 100 nm (bottom), core/shell fibre images—10 μm (left) and 100 nm (right), and electrolyte image—1 μm, ( c ), cell voltage and power density as functions of current density and ( d ), a typical impedance spectrum measured under open circuit conditions. The tests were carried out at 550 °C. Air was supplied to the cathode (300 ml min −1 ) and H 2 was supplied to the anode (80 ml min −1 ). Full size image Table 2 Single-cell tests. 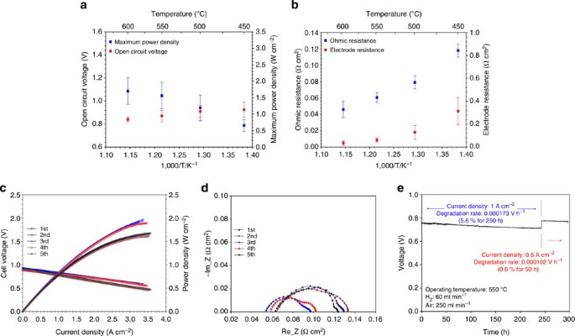Figure 6: Reproducibility and durability of the GDC-based LT-SOFC. Performance obtained from the core/shell-fibre-structured Ba0.5Sr0.5Co0.8Fe0.2O3−δ-Gd0.1Ce0.9O1.95(~30 μm) | Gd0.1Ce0.9O1.95(~5 μm) | nanocomposite Ni-Gd0.1Ce0.9O1.95anode functional layer (~10 μm) | Ni-Gd0.1Ce0.9O1.95(~800 μm) fuel cell at different temperatures. Air was supplied to the cathode (300 ml min−1) and H2was supplied to the anode (80 ml min−1). (a), OCVs and maximum power densities as a function of temperature on the multiple cell tests (Error bars indicate s.d. of the results based on the multiple tests under the same conditions.) (b), ohmic and electrode ASRs as a function of temperature on the multiple cell tests (Error bars indicate s.d. of the results based on the multiple tests under the same conditions.) (c), cell voltage and power density as functions of current density in the five times multiple tests at 550 °C, (d), impedance spectra on the five times multiple tests at 550 °C under open circuit conditions, and (e), short-term test at 550 °C. Air was supplied to the cathode (250 ml min−1), and H2was supplied to the anode (60 ml min−1). Full size table Reproducibility and durability of the GDC-based LT-SOFC Figure 6a–d show the results of the multiple cell tests to confirm the reproducibility of the GDC-based LT-SOFCs. The peak power densities were about 1.705±0.405, 1.562±0.405, 1.192±0.391 and 0.655±0.185 W cm −2 at 600, 550, 500 and 450 °C, respectively ( Fig. 6a ). The ASRs ohmic were approximately 0.046±0.01, 0.060±0.006, 0.079±0.008 and 0.118±0.008 Ω cm 2 at 600, 550, 500 and 450 °C and the ASRs electrode were approximately 0.035±0.019, 0.061±0.018, 0.129±0.060 and 0.314±0.119 Ω cm 2 at 600, 550, 500 and 450 °C, respectively ( Fig. 6b ). The majority of the cells showed approximately 1.7–1.9 W cm −2 of the maximum power density at 550 °C, but one or two tests produced large deviations, which could be attributed to the low OCV (0.84–0.85 V at 500 °C). Although the OCV should increase with a decrease in the operating temperature, the OCVs of the cells barely increased with the decrease in the temperature, which agrees with the results reported by Ding et al. [54] : 0.85 V (2 μm) and 0.96 V (4 μm) at 500 °C. Most of the cells had uniform and thin electrolytes with a thickness of 5–6 μm, but undesired dents appeared in the low OCV cells. The section where the electrolyte subsided was only 3 μm in thickness ( Supplementary Fig. 9 ). The raw I–V curves and impedance spectra obtained from the typical five times cell tests clearly prove that the GDC-based LT-SOFCs had the reproducible performance at 550 °C, showing about 1.8±0.1 W cm −2 (a margin of error of about only 5%) in a maximum power density and about 0.058±0.004 Ω cm 2 and 0.051±0.008 Ω cm 2 in the ASRs ohmic and ASRs electrode , respectively ( Fig. 6c,d ). For that reason, we believe that the high-performance GDC-based LT-SOFCs are reproducible in this study. Figure 6: Reproducibility and durability of the GDC-based LT-SOFC. Performance obtained from the core/shell-fibre-structured Ba 0.5 Sr 0.5 Co 0.8 Fe 0.2 O 3− δ -Gd 0.1 Ce 0.9 O 1.95 (~30 μm) | Gd 0.1 Ce 0.9 O 1.95 (~5 μm) | nanocomposite Ni-Gd 0.1 Ce 0.9 O 1.95 anode functional layer (~10 μm) | Ni-Gd 0.1 Ce 0.9 O 1.95 (~800 μm) fuel cell at different temperatures. Air was supplied to the cathode (300 ml min −1 ) and H 2 was supplied to the anode (80 ml min −1 ). ( a ), OCVs and maximum power densities as a function of temperature on the multiple cell tests (Error bars indicate s.d. of the results based on the multiple tests under the same conditions.) ( b ), ohmic and electrode ASRs as a function of temperature on the multiple cell tests (Error bars indicate s.d. of the results based on the multiple tests under the same conditions.) ( c ), cell voltage and power density as functions of current density in the five times multiple tests at 550 °C, ( d ), impedance spectra on the five times multiple tests at 550 °C under open circuit conditions, and ( e ), short-term test at 550 °C. Air was supplied to the cathode (250 ml min −1 ), and H 2 was supplied to the anode (60 ml min −1 ). Full size image A short-term test was carried out on the GDC-based LT-SOFC to verify the durability and the structural stability. On the basis of the high maximum power density at low temperatures, a high current density of 1 A cm −2 was applied to the GDC-based LT-SOFC. Figure 6e shows the stability of the GDC-based LT-SOFC at a current density of 1 A cm −2 starting at 0.756 V for approximately 250 h and, thereafter, at a current density of 0.5 A cm −2 starting from 0.776 V for the next 50 h. Considering that the unmodified GDC-based cells commonly show 0.7 V at 0.3–0.4 A cm −2 , the tailored GDC-based LT-SOFCs can reduce the number of unit cells required for SOFC stacks, which would be beneficial for the auxiliary power units in automobiles. The voltage degradation was approximately 5.6% over 250 h with a degradation rate of 0.00017 V h −1 . Hagen et al. [55] reported that the voltage degradation was fairly linear at lower current densities, and it was more exponential at higher current densities. However, although the high current density of 1 A cm −2 was applied, the GDC-based LT-SOFC was stable for the tested time period of approximately 250 h. Compared with the voltage degradation rates between the applied current densities of 1 and 0.5 A cm −2 , less voltage degradation occurred under the latter conditions. The voltage degradation at 0.5 A cm −2 was approximately 0.6% over 50 h with a degradation rate of 0.00010 Vh −1 . These results show that stable and high performance at low temperatures can be obtained using the GDC-based LT-SOFC in a configuration of the core/shell fibre-structured BSCF-GDC cathode | GDC electrolyte (5 μm) | nanocomposite Ni-GDC AFL | Ni-GDC anode. In summary, the GDC-based LT-SOFC in configuration of the core/shell fibre-structured BSCF-GDC cathode (~30 μm) | GDC electrolyte (5 μm) | nanocomposite Ni-GDC AFL (~10 μm) |Ni-GDC anode (~800 μm) was prepared, which showed a high performance of approximately 2 W cm −2 at 550 °C in hydrogen. It could be attributed to the decrease in both the ohmic loss and the activation loss, resulting from a combination of the thin GDC electrolyte, the nanocomposite AFL and the core/shell fibre-structured BSCF-GDC cathode. The GDC thin electrolyte was successfully deposited on the AFL using the cost-effective dip-coating method. The nanocomposite AFL and the core/shell-fibre-structured BSCF-GDC cathode had reproducible structures. Particularly, the core/shell-fibre-structured BSCF-GDC cathode via the AE&P process significantly reduced the activation losses at low temperatures. Nearly all the tailored GDC-based LT-SOFCs were reproducible and stable for 300 h even under the high current density of 1 A cm −2 . These results allude to the possibility that the stable- and high-performance LT-SOFCs can be achieved simply by modifying the microstructures of the SOFC components based on the traditional cell configurations. Therefore, we suggest that the original cell design of the core/shell-fibre-structured Ba 0.5 Sr 0.5 Co 0.8 Fe 0.2 O 3−δ -Gd 0.1 Ce 0.9 O 1.95 cathode | thin Gd 0.1 Ce 0.9 O 1.95 electrolyte | nanocomposite Ni-Gd 0.1 Ce 0.9 O 1.95 AFL | Ni-Gd 0.1 Ce 0.9 O 1.95 anode can not only be a good guide for the fabrication of stable and high-performance LT-SOFCs but also benefit the development of the LT-SOFCs. Nanocomposite Ni-GDC AFL Nanocomposite Ni-GDC AFL powders were prepared using the Pechini [34] . The AFL powders (10 g) calcined at 600 °C were ball-milled with EFKA 4340 (0.4 ml) as a dispersant in a mixed toluene/isopropyl alcohol (IPA; 100 ml) for 12 h. Thereafter, Di- n butylphthalate (2 ml) as a plasticiser, Triton-X (0.4 ml) as a surfactant and polyvinyl butyral (0.5 g) as a binder were added to the suspension, and then the AFL slurry was ball-milled for 24 h. GDC thin electrolyte To reduce the GDC electrolyte thickness through a dip-coating process, we manipulated the compositions of the electrolyte slurries. Commercial Gd 0.1 Ce 0.9 O 1.95 powders with surface areas of 10–14 m 2 g −1 and particle sizes (d50) of 0.1–0.4 μm (GDC, Fuel cell materials) were used as an electrolyte material. The GDC powders were ball-milled with EFKA 4340 as a dispersant in a mixed toluene/IPA for 12 h. Next, Di-n butylphthalate as a plasticiser, Triton-X as a surfactant and polyvinyl butyral as a binder were added to the suspension, and then the GDC slurry was ball-milled for 24 h. The slurries 1, 2 and 3 were different in the amount of the GDC powders and toluene/IPA solvent ( Supplementary Table 3 ). The viscosities of the slurries decreased with a decrease in the amount of the GDC powder, reaching approximately 5.3±0.1, 2.5±0.1 and 2.3±0.1 cP at 100 r.p.m. in slurries 1, 2 and 3, respectively ( Supplementary Fig. 10 ). The dip-coating process was carried out on the anode supports without the AFL. When slurries 1, 2 and 3 were used in the dip-coating process, the GDC electrolyte thicknesses were approximately 13, 7 and 3 μm, respectively. The minimum thickness throughout the dip-coating process was approximately 3 μm. However, the electrolytes of the GDC-based LT-SOFCs were fabricated using slurry 2 due to the obscurity of the interface between the 3-μm-thick electrolyte and the anode support. BSCF fibre cores The advanced electrospinning based (AE) on dispersed particles, which was developed in our previous research [43] , was carried out in this study. Ba 0.5 Sr 0.5 Co 0.8 Fe 0.2 O 3− δ powder (Kceracell, S BET =5–10 m 2 g −1 , PSD (d50)=0.3–0.6 μm) and poly vinyl pyrrolidine (PVP average ≈1,300,000, Sigma Aldrich) were mixed in ethanol under vigorous stirring for 1 h. The weight ratios of PVP to ethanol and PVP to the BSCF powders were 1:10 and 1:1, respectively. The viscosity of completely dissolved PVP/ethanol solution was 100–150 cP. The viscous suspension for electrospinning was injected using a syringe with a thin needle (30 G, 0.15 mm inner diameter) at a constant rate of 30 μl min −1 . An electric field of 15 kV was applied between a collector and needle tip, sustaining a temperature of 20 °C and humidity of 35%. The PVP-BSCF nanowires were calcined at 500 °C for 6 h in an air atmosphere at a heating rate of 1 °C min −1 . BSCF-GDC core/shell fibres The BSCF-GDC core/shell fibres were prepared using the Pechini method. Gd(NO 3 ) 3 ·6H 2 O (Sigma Aldrich) and Ce(NO 3 ) 3 ·6H 2 O (Sigma Aldrich) were used as metal precursors. First, Gd(NO 3 ) 3 ·6H 2 O and Ce(NO 3 ) 3 ·6H 2 O were dissolved in distilled water with molar fractions of 0.1:0.9. After stirring for 3 h at room temperature, citric acid (CA; Duksan) and ethylene glycol (EG; Sigma Aldrich) were added into the solution containing the metal salts (M) ([CA]/[M]=1 and [EG]/[CA]=4). The calcined BSCF fibre cores were added into the GDC solution, and then vigorous stirring was carried out at 70 °C. The weight ratio of the BSCF fibre cores to the GDC shell particles is 7:3. The polymeric sol was burned out at 200 °C to obtain the BSCF-GDC core/shell fibres. The core/shell fibres were calcined at 600 °C for 3 h. The core/shell fibre-structured BSCF-GDC powders were fabricated to the cathode paste. To compare with the BSCF-GDC core/shell fibre cathode in the symmetrical cell tests, the conventional BSCF-GDC powders were prepared by ball-milling in ethanol with the same weight ratio as the BSCF-GDC core/shell fibres. Ba 0.5 Sr 0.4 Co 0.8 Fe 0.2 O 3− δ (Kceracell, S BET =5–10 m 2 g −1 , PSD (d50)=0.3–0.6 μm) powders and Gd 0.1 Ce 0.9 O 1.95 (Rhodia, ULSA grade) powders with surface area of <10 m 2 g −1 and particle size (d50) of about 1 μm were used as the materials for the conventional BSCF-GDC cathode. The conventional BSCF-GDC powders were fabricated into the cathode paste. Symmetrical cells Gd 0.1 Ce 0.9 O 1.95 (Fuel cell materials) was used as an electrolyte material. GDC powders were pressed under 98 MPa to form disk-like pellets with diameters of 3.6 cm and thicknesses of 1.5 mm. The electrolyte supports were sintered at 1500 °C for 5 h. The BSCF-GDC core/shell fibre cathode and conventional BSCF-GDC cathode pastes were coated on the both side of the electrolyte surfaces by screen-printing method. All symmetrical cells were sintered at 950 °C for 2 h. GDC-based LT-SOFCs NiO (99%, J. T. Baker), Gd 0.1 Ce 0.9 O 1.95 powders (Rhodia, ULSA grade; 60:40 by weight) and a carbon black (10 wt. % for the NiO-GDC powder) were ball-milled in ethyl alcohol (99.9%, Duksan Pure Chemical) to fabricate Ni-GDC anode supports. The NiO-GDC powders were dried at 80 °C for 24 h and pressed under 88 MPa. The disk-like NiO-GDC anodes with diameter of 3.6 cm and thickness of 1.5 mm were partially sintered at 1,100 °C for 3 h. The nanocomposite AFL slurry was coated on the disk-like NiO-GDC anode supports by dip-coating method to make the second generation cells. The dip-coating process was carried out once for the AFL. The holding time is 15 s, and the velocity at which the anode support layer was removed from the slurry is 1.6 mm s −1 . The anode supports with the AFL were sintered at 1,100 °C for 3 h. The prepared GDC electrolyte slurry 2 was coated on the AFL using a dip-coating method, and then the half-cells were fully sintered at 1500 °C for 3 h. The electrolyte coating was carried out three times at the same condition as the AFL coating. The anode side of the half-cells was polished to a thickness of 800 μm. The core/shell fibre cathode paste was coated on the electrolyte side of the half-cells using a screen-printing method, and then the cells were sintered at 950 °C for 2 h. The first generation cells were prepared by the same procedures as the second generation cells except the AFL coating. The complete cells had approximately 800 μm in the anode thickness and 2.6 and 1 cm in the anode and cathode diameters, respectively. Characterizations The crystal structures of the BSCF-GDC core/shell fibres were measured by X-ray diffractometer (Rigaku, Miniflex model) with Cu Kα radiation at room temperature. The weight loss and heat flow of the BSCF-GDC core fibres and BSCF core/shell fibres were detected in a temperature range from 100 to 1000 °C in air atmosphere by thermogravimetric analysis and differential scanning calorimeter (Mettler Toledo, 1100 SF) before the calcination process. Field Emission Scanning Electron Microscopy (FE-SEM) (JSM-7001F) equipped with EDX (FE-SEM, JEOL, JSM-7001F model) was used to observe the morphologies and compositions of the BSCF-GDC core/shell fibres, the GDC-based LT-SOFC and each component. Field emission transmission electron microscopy (FE-TEM or HRTEM; JEOL, JEM 2100-F model) was used to distinguish the GDC shell nanoparticles from the BSCF core fibres. The specific surface area of the BSCF-GDC particles and core/shell fibres calcined at 950 °C for 2 h were measured by Brunauer–Emmett–Teller (BET) isotherm technique with nitrogen adsorption using a surface area analyser (BELSORP mini-II, BEL Japan, Inc.). The symmetrical cell tests were carried out between 450 and 600 °C under an air atmosphere. The single-cell tests were also conducted between 600 and 450 °C under the following conditions: air was supplied to the cathode (300 ml min −1 ) and H 2 was supplied to the anode (80 ml min −1 ). Pyrex ring and Pt paste were used as a sealant and current collector, respectively. A FC Impedance metre (Kikusi, KFM 2030) and versatile multichannel potentiostat (Biologic, VMP3B-10) were used for the electrochemical analysis of the GDC-based LT-SOFCs. The impedance spectra were measured in a frequency range from 0.1 to 1 MHz with signal amplitude of 10 mV rms under open circuit condition. The short-term test was carried out at 550 °C at a current density of 1 A cm −2 and the following conditions: air was supplied to the cathode (250 ml min −1 ) and H 2 was supplied to the anode (60 ml min −1 ). How to cite this article: Lee, J. G. et al. Tailoring gadolinium-doped ceria-based solid oxide fuel cells to achieve 2 W cm −2 at 550 °C. Nat. Commun. 5:4045 doi: 10.1038/ncomms5045 (2014).